Structural domain walls in polar hexagonal manganites The domain structure in the multiferroic hexagonal manganites, h- R MnO 3 ( R =Sc, Y, Dy-Lu), is currently intensely investigated, motivated by the observation of nanoscale electrical conductivity at the domain walls and intriguing sixfold topological defects at their meeting points, as well as reports of coupling between ferroelectricity, magnetism and structural antiphase domains. The detailed structure of the domain walls, as well as the origin of such couplings, however, was previously unknown. Here we use first-principles electronic structure calculations to elucidate the structure and properties of the structural domain walls in the hexagonal manganites. Our results allow us to explain why ferroelectric domain walls are always simultaneously antiphase walls, propose a mechanism for ferroelectric switching through domain-wall motion, suggest a structure for the observed sixfold topological defects and predict a topological protection of experimentally observed stripe domains in hexagonal manganites. In ferroic materials such as ferroelectrics, regions that differ in the orientation of the ferroic order parameter—the electrical polarization in ferroelectrics—are called domains. The planar defects that form between adjacent domains are then domain walls (DWs). In general, DWs have a different symmetry and structure than the bulk of the domains, and have an important role in the switching mechanism of the associated order parameter. In multiferroic materials, which contain multiple simultaneous ferroic orders, the DWs are of particular interest. For example, the ferroelectric DWs in multiferroics have been shown to exhibit novel properties such as local conduction [1] , [2] , [3] , [4] and local magnetization [5] . In addition, couplings among multiple (anti-)ferroic orders, which are not observed in the bulk systems, have been reported at the DWs [6] , [7] , [8] . The hexagonal manganites h- R MnO 3 ( R =Sc, Y, Dy-Lu) ( Fig. 1 ), with their coexisting ferroelectricity ( T C ≈1,200–1,500 K) and antiferromagnetism ( T N ≈70–130 K), are currently among the most intensely investigated multiferroics [6] , [9] , [10] , [11] . They are improper geometric ferroelectrics, in which the primary order parameter is a structural tilt trimerization of the MnO 5 polyhedra, which is driven by minimization of the electrostatic energy [11] , [12] , [13] . The trimerization corresponds to the condensation of a zone-boundary K 3 mode of the high-symmetry P 6 3 / mmc structure, and lowers the symmetry to the polar P 6 3 cm space group [12] , [14] , but does not itself introduce a net ferroelectric polarization. The trimerization is characterized by two angles: the angle θ between the z axis and the Mn-apical O bond gives the magnitude of the tilting and can be regarded as the order parameter of the K 3 mode ( Fig. 1c ), and an azimuthal angle, φ , which describes the orientation of the tilting. Below the phase transition φ adopts one of six values separated by 60°, which correspond to trimerization around three possible origins, with in- or out-orientation of the tilting; as a result six structural domains emerge, as shown in Fig. 2a (refs 14 , 15 , 16 ). The polar mode emerges as a result of an anharmonic coupling with the K 3 mode [12] , and the orientation of the subsequent ferroelectric polarization is set by the in- or out-orientation of the K 3 tilting [14] . Then, φ =0°, 60°, 120°, 180°, 240° and 300° are often labelled α + , β − , γ + , α − , β + and γ − ( Fig. 2a ), where α, β and γ represent different origins for the trimerization, and + or − indicate the out- or in-orientation of the tilts and correspondingly the up- or down-orientation of the ferroelectric polarization. 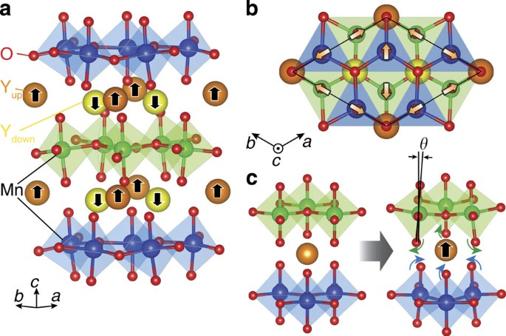Figure 1: Crystal structure of hexagonal manganites. The structure is shown perpendicular (a,c) and along (b) thecaxis. The directions of displacements of the Y ions are indicated by the black arrows and the yellow (down) or orange (up) colours; Mn ions in successive layers, and their associated polyhedra, are coloured blue or green, respectively. The yellow arrows inbshow the direction of displacement of the apical oxygen ion associated with the polyhedral tilting. In panelcthe effect of theK3trimerization from the paraelectric phase (left) on theRion and its surrounding MnO5trigonal bipyramids is shown;θis the tilting magnitude. Note that the tilt pattern and the direction of theRion displacement are determined by the origin of the trimerization and the in- or out-orientation of the tilts. Figure 1: Crystal structure of hexagonal manganites. The structure is shown perpendicular ( a , c ) and along ( b ) the c axis. The directions of displacements of the Y ions are indicated by the black arrows and the yellow (down) or orange (up) colours; Mn ions in successive layers, and their associated polyhedra, are coloured blue or green, respectively. The yellow arrows in b show the direction of displacement of the apical oxygen ion associated with the polyhedral tilting. In panel c the effect of the K 3 trimerization from the paraelectric phase (left) on the R ion and its surrounding MnO 5 trigonal bipyramids is shown; θ is the tilting magnitude. Note that the tilt pattern and the direction of the R ion displacement are determined by the origin of the trimerization and the in- or out-orientation of the tilts. 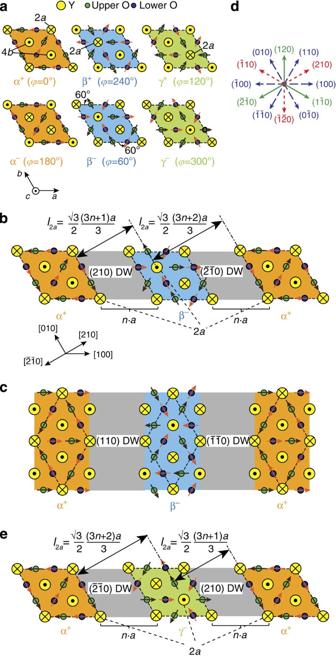Figure 2: Definition of DWs in hexagonal manganites. (a)Schematics of the six possible structural domains in YMnO3. The view is along thecaxis, parallel to the direction of ferroelectric polarization. The large yellow circles show the positions of Y ions, with crosses or dots indicating displacement into or out of the plane. The small circles are the adjacent oxygens at the apices of the trigonal bipyramids, with arrows indicating the direction of their displacements from the high-symmetryP63/mmcphase. We label each domain by its phaseφ, defined to be the (counter)clockwise angle of the displacement directions of upper (lower) oxygens relative to those in the α+domain14. (b,c) Our nomenclature for the neutral DWs sandwiched between α+and β−domains. The (210) andDWs are inequivalent that can be seen by comparing the spacing between the 2aWykoff positions,, which are different in each antiphase domain:a(wherenis an integer) across a (210) DW andaacross aDW. In contrast the (110) andDWs are equivalent by symmetry (see text for details). (d) Classification of DWs according to the normal vector (arrows) connecting an α+to a β−domain. Equivalent DWs are drawn with the same colour. (e) DWs between α+and γ−domains. Note that the (210) andDWs are reversed relative to those between α+and β−domains. Full size image Figure 2: Definition of DWs in hexagonal manganites. ( a )Schematics of the six possible structural domains in YMnO 3 . The view is along the c axis, parallel to the direction of ferroelectric polarization. The large yellow circles show the positions of Y ions, with crosses or dots indicating displacement into or out of the plane. The small circles are the adjacent oxygens at the apices of the trigonal bipyramids, with arrows indicating the direction of their displacements from the high-symmetry P 6 3 / mmc phase. We label each domain by its phase φ , defined to be the (counter)clockwise angle of the displacement directions of upper (lower) oxygens relative to those in the α + domain [14] . ( b , c ) Our nomenclature for the neutral DWs sandwiched between α + and β − domains. The (210) and DWs are inequivalent that can be seen by comparing the spacing between the 2 a Wykoff positions, , which are different in each antiphase domain: a (where n is an integer) across a (210) DW and a across a DW. In contrast the (110) and DWs are equivalent by symmetry (see text for details). ( d ) Classification of DWs according to the normal vector (arrows) connecting an α + to a β − domain. Equivalent DWs are drawn with the same colour. ( e ) DWs between α + and γ − domains. Note that the (210) and DWs are reversed relative to those between α + and β − domains. Full size image These recent studies have raised many intriguing questions regarding the nature of the DWs. First, while three types of structural DWs—ferroelectric only (FE), antiphase only (AP) and antiphase plus ferroelectric (AP+FE)—might be expected, only AP+FE DWs have been observed [15] , [16] . Detailed scanning transmission electron microscopy (STEM) studies [17] of these AP+FE DWs, however, have not converged to a single structural model of the lowest energy structure. Second, no model for evolution of the ferroelectricity—which in this case is not the primary ferroic order parameter—through motion of the coupled AP+FE DWs exists, although first-principles calculations have shown that ferroelectric switching in the absence of DW motion is prohibitive [18] . Finally, the structure of the topologically protected sixfold defects formed at the intersections of AP+FE DWs [4] , [5] , [13] , [15] , [16] , [19] , [20] is unknown. In this work, we present a detailed systematic study of the structures and energetics of neutral DWs in YMnO 3 using first-principles density functional theory in order to contribute to answering these questions. Definition of DWs We begin by introducing our nomenclature for the neutral DWs in h-YMnO 3 . We first consider DWs between α + and β − domains. We define the (210) DW to be the wall for which the normal vector from an α + domain to a β − domain points along the (210) direction with respect to the primitive unit cell vectors ( Fig. 2b , left wall). The DW is then the wall with the same orientation, but with the α + and β − domains reversed, as shown on the right of Fig. 2b . The structures, and therefore in principle the energetics, of the (210) and DWs are in fact different, as can be seen for example by comparing the distances, , between the layers of Y ions at the 2 a Wyckoff position [21] across the wall ( Fig. 2b ). On the other hand, the , and (210) DWs (normal vector from α + to β − pointing along ( 0), ( 10) and (210) directions) are all equivalent to each other by symmetry, and the (120), and DWs (defined analogously) also form a symmetry-equivalent set. We refer to these two types of DWs as {210} and {120} DWs, respectively. Finally, the two DWs perpendicular to the [110] direction—(110) and DWs ( Fig. 2c )—are identical by symmetry and equivalent also to (100), (010), and DWs. We refer to this type as {110} DWs. The equivalent DWs between α + and β − domains are collected in Fig. 2d . The DWs between β + and γ − , and between γ + and α − are equivalent to that between α + and β − , for the same DW direction. Furthermore, the DW between α − and β + is equivalent to that between α + and β − because of the m z symmetry operation. α + to γ − is however the reverse of α + to β − ( Fig. 2e ). Theoretical calculations on neutral DWs Our first task is to calculate the structure of the lowest energy neutral DWs. As a starting point to construct our supercells, we take the DW models proposed by Choi et al. [15] . These have the orientation of the {120} and {210} DWs in our nomenclature, and are obtained by averaging the structures of two neighbouring domains so that the Y ions along the wall retain the high-symmetry positions of the paraelectric phase. Such a model is physically reasonable as walls that are the structural average of two different domains, and which, therefore, retain aspects of the paraelectric structure, are known to be stable in perovskite-structure ferroelectrics [22] , [23] , [24] . In our calculations, however, we remove the symmetry constraint by slightly displacing the Y ions at the DWs along z direction, and fully relax all internal positions. In our structurally optimized walls, shown in Fig. 3a , the Y ions in fact do not occupy their high-symmetry sites, but instead change abruptly from one displacement pattern to another, so that the DWs have twofold screw rotation and c -glide reflection symmetries. In the three panels of Fig. 3a , we show the calculated Mn-O distances, θ and φ angles, and local polarizations obtained from (where e is the electron charge, Ω is the volume of a single unit cell, u is the displacement of atom α in the z direction from its paraelectric position, and Z α are the formal charges) summed over three adjacent layers. Dashed lines indicate the bulk quantities, which are recovered at the middle of each domain. We find that φ , θ and the local polarization change abruptly across the DW from one bulk value to the next, and we can consider the DW width to be effectively zero; we refer to them subsequently as sharp DWs. Note that the apparent slightly higher local polarizations near the DWs are caused by the different up/down displacement patterns of the Y ions from the bulk, and our choice of averaging over three layers. In addition, the Mn-O bond lengths remain unchanged across the DWs, indicating that the polyhedra retain their bulk shape. Note that if we define the microscopic DW to be the point at which the structural phase φ changes abruptly, we find that the {210} and {120} DWs zigzag when viewed along the c axis (black dashed lines in Fig. 3a ), and have length times longer than the corresponding DWs that would be observed in mesoscopic experiments such as piezoresponse force microscopy (PFM). The wall width is much thinner than expected for a ferroelectric DW, which is typically a few unit cells wide, but rather characteristic for an antiphase boundary. In Fig. 3b we plot the average DW energy as a function of DW spacing (achieved by varying the supercell size), and find only a weak dependence, indicating that adjacent walls are neither strongly repulsive nor attractive. Our calculated average sharp DW energy extrapolated to infinite spacing is 11.2 mJ m −2 . Note that the supercells considered above contain both a {120} and a {210} DW, and the calculated DW energy is the average value. To extract individual DW energies, we constructed supercells containing only one type of DW ( Supplementary Fig. S1 ). Our results are shown as the stars and squares in Fig. 3b ; we find that the {210} sharp DW is in fact lower energy. The Y ions displace in an up-down-up-down pattern across the {210} DWs, and an up-up-down-down pattern across {120} DWs ( Fig. 3a ), which likely contributes to differences in the electrostatic energies. Local electronic structure at the DWs is shown in Supplementary Fig. S2 and discussed in Supplementary Note S1 . 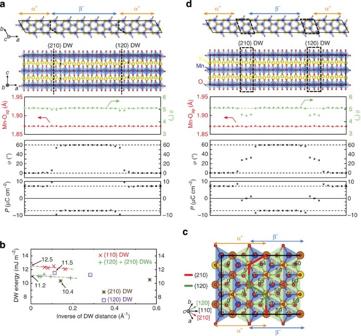Figure 3: Calculated DWs in YMnO3. {120} and {210} DW structures (upper panels) for (a) the sharp models and (d) the 2/cDW models. The dashed lines in the sharp models show the position of the DW, defined by the abrupt change in the phaseφ. The lower panels show the average Mn-apical O distance, the tilting magnitude (θ) and phase angle (φ) of the MnO5bipyramids and the local layer polarization,P. Dashed lines indicate the bulk quantities, which are recovered in the middle of each domain. (b) Energies for {110}, {120} and {210} DWs calculated with different supercell sizes. The dash-dotted lines are linear extrapolations to infinite spacing (zero inverse distance). Plus signs (+) indicate the averages of {120} and {210} DW energies calculated with the supercells containing both DWs. (c) Calculated {110} DW structure for the sharp model with a 300-atom supercell. Only half of the supercell is shown. The numbers are the averageφvalue at each column of MnO5bipyramids, and the thick line indicates the {110} DW separating the α+domain withφ~0° and the β−domain withφ~60°. We see that the {110} DW can be regarded as a combination of {120} and {210} DWs. Figure 3: Calculated DWs in YMnO 3 . {120} and {210} DW structures (upper panels) for ( a ) the sharp models and ( d ) the 2/ c DW models. The dashed lines in the sharp models show the position of the DW, defined by the abrupt change in the phase φ . The lower panels show the average Mn-apical O distance, the tilting magnitude ( θ ) and phase angle ( φ ) of the MnO 5 bipyramids and the local layer polarization, P . Dashed lines indicate the bulk quantities, which are recovered in the middle of each domain. ( b ) Energies for {110}, {120} and {210} DWs calculated with different supercell sizes. The dash-dotted lines are linear extrapolations to infinite spacing (zero inverse distance). Plus signs (+) indicate the averages of {120} and {210} DW energies calculated with the supercells containing both DWs. ( c ) Calculated {110} DW structure for the sharp model with a 300-atom supercell. Only half of the supercell is shown. The numbers are the average φ value at each column of MnO 5 bipyramids, and the thick line indicates the {110} DW separating the α + domain with φ ~0° and the β − domain with φ ~60°. We see that the {110} DW can be regarded as a combination of {120} and {210} DWs. Full size image Our finding that the width of the lowest energy DW is effectively zero is in contrast to the behaviour in conventional perovskite counterparts such as PbTiO 3 , where the widths of 180° DWs are narrow but finite (≥1 unit cell width) [22] , [23] , [24] , and the ions in the wall region transition from one orientation to the other through their high-symmetry paraelectric positions. The adoption of the high-symmetry position in conventional ferroelectrics can be regarded as a geometric frustration of the positions in the two opposite domain structures. This frustration does not exist in h-YMnO 3 , because the displacement patterns of the Y ions, determined by the tiltings of the MnO 5 trigonal bipyramids, can be locally preserved through the DWs, as seen in Fig. 3a . Instead, the translational periodicity that is broken at the DWs is reminscent of stacking faults commonly observed in close-packed structures. It is also interesting to note that the 180° DW energy in YMnO 3 is considerably lower than those of perovskites with similar Curie temperatures, for example the corresponding 180° DW energy in PbTiO 3 ( T C =765 K) is 132 mJ m −2 ( [22] ) and in BiFeO 3 ( T C =1,100 K) it is between 80 and 800 mJ m −2 , depending on the treatment of the oxygen rotations [23] , [25] . While in conventional ferroelectrics, Curie temperatures often correlate with the magnitude of the ferroelectic polarization, this is not the case in YMnO 3 where the Curie temperature determined by the tilt transition [12] is high (1,258±14 K) (ref. 21 ), while the improper ferroelectric polarization is not large (5.6 μC cm −2 ). Winding DWs Experimentally, most DWs do not form straight lines corresponding to a single orientation, and so for comparison we next calculate the structure and energetics of the set of {110} DWs. Figure 3c shows our relaxed {110} DW structure calculated within a 300-atom supercell, which was initialized by displacing the Y ions along the z axis to create sharp DWs in the manner of our lowest energy {120} and {210} DWs. This sharp configuration is retained on fully relaxing the supercell, and again our calculated lowest energy DW width is effectively zero. Since the {110} and DWs are symmetry equivalent for this wall orientation, we can extract their energies directly from supercells containing both walls. Our calculated extrapolated infinite-separation DW energy is 12.5 mJ m −2 ( Fig. 3b ), which is slightly higher than those of {120} and {210} DWs. In fact the {110} DW can be regarded as a combination of {120} and {210} DWs ( Fig. 3b ), and indeed the {110} DW energy estimated from the {120} and {210} DW energies is mJ m −2 , which is close to our explicitly calculated value. Microscopically, the length of the {110} DW line set by the change in φ (solid red and green line in Fig. 3c ) is 4/3=1.33 times longer than that of the straight DW. It is clear from the schematic in Fig. 4a that a general winding DW can be decomposed into contributions from {120} (green), {210} (red) and {110} (blue) DWs, with the latter being combinations of {120} and {210} DWs. The energy of a DW pointing in an arbitrary direction can then be estimated from the geometrical relations given in Fig. 4b . Our finding that the {210} DW has the lowest energy explains the recently observed stripe domain patterns in h- R MnO 3 grown below the trimerization temperatures [20] . The authors of [20] report that the stripe lines lie along the 110 directions. The DWs perpendicular to the [110] direction are or (see Fig. 2d ), which belong to our low-energy {120} and/or {210} sets, respectively. From our results, we suggest that the DWs are likely to be of {210} type. As two {210} DWs do not annihilate on contact, we expect a topological protection of the stripe domains under electric-field application even without the presence of sixfold topological defects. We note that it has been shown using Landau theory [14] that the lowest-order coupling of the inhomogeneous trimerisation to strains causes such stripe domains to be the topologically stable ground state in the presence of uniaxial strain. 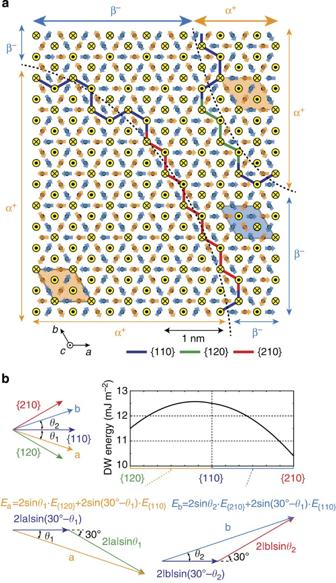Figure 4: Structure and energetics of winding DWs. (a) Schematics of winding AP+FE DWs, which are combinations of {120}, {210}, and {110} DWs. The dashed lines indicate the position of a mesoscopically observed DW with the directions of Y ion displacements changed on either side of the wall. The thick lines indicate the DWs derived from the change in tilt angle of the MnO5polyhedra. (b) DW energy as a function of the DW direction, which is geometrically interpolated from our calculated {120}, {210} and {110} DW energies,E{120},E{210}, andE{110}. Figure 4: Structure and energetics of winding DWs. ( a ) Schematics of winding AP+FE DWs, which are combinations of {120}, {210}, and {110} DWs. The dashed lines indicate the position of a mesoscopically observed DW with the directions of Y ion displacements changed on either side of the wall. The thick lines indicate the DWs derived from the change in tilt angle of the MnO 5 polyhedra. ( b ) DW energy as a function of the DW direction, which is geometrically interpolated from our calculated {120}, {210} and {110} DW energies, E {120} , E {210} , and E {110} . Full size image AP and FE DWs Next we perform structural relaxations for AP-only and FE-only DWs, to understand microscopically why such walls do not occur in h- R MnO 3 . Based on our results for the AP+FE DWs, we constructed initial models that preserve the up-up-down or down-down-up displacements of the Y ions through the DWs. As shown in Fig. 5 , the subsequently relaxed structures retain the off-centering of the Y ions. By analysing the tilt patterns of the MnO 5 polyhedra, and the corresponding Y off-centering patterns, we see that an AP-only DW is in fact an atomic-scale composite of two AP+FE DWs. Likewise a FE-only DW is an atomic-scale composite of three AP+FE DWs. Indeed, the average DW energies that we obtain for AP-only and FE-only DWs with 270- and 300-atom supercells are 23.0 and 34.4 mJ m −2 , respectively; almost exactly two and three times the average value for the AP+FE DWs (11.2 mJ m −2 ). This is consistent with the recent Landau theory analysis [14] , which showed that AP+FE DWs change the phase by only ±60°, whereas the phase difference between two domains with different origin is 120°, and that between two domains with different polarization is 180°. We also mention that our calculated DW energies are not consistent with the six-state clock model used in [20] for Monte Carlo simulation, in which the ratio of AP+FE, AP-only and FE-only DW energies was assumed to be 1:3:4. 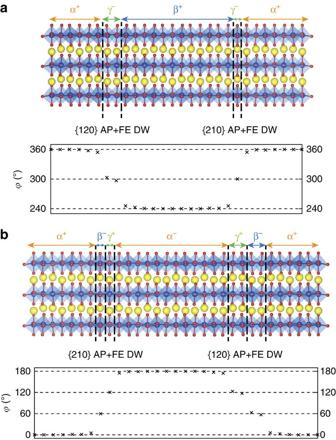Figure 5: AP and FE DWs. Calculated (a) AP and (b) FE DWs perpendicular to the [210] axis with 270- and 300-atom supercells, respectively. The relaxed structures locally preserve the up-up-down or down-down-up displacements of the Y ions across the DWs, resulting in the intermediate domains. Figure 5: AP and FE DWs. Calculated ( a ) AP and ( b ) FE DWs perpendicular to the [210] axis with 270- and 300-atom supercells, respectively. The relaxed structures locally preserve the up-up-down or down-down-up displacements of the Y ions across the DWs, resulting in the intermediate domains. Full size image Interestingly, our calculations show that the intermediate domains that invariably exist at FE-only and AP-only DWs can be as narrow as or , depending on the phase difference between the domains. We note, however, that our density functional theory (DFT) calculations are performed at 0 K, and the absence of AP-only and FE-only walls is likely due to an entropy-driven decomposition of the atomic-scale wall composites. As the system cools through the trimerization temperature (1,258±14 K), the formation of domains with all allowed choices of phase will naturally result in some AP-only and FE-only walls. However, as these walls are composites of AP+FE walls, they would likely decompose due to entropy at high temperature because (i) the wall energy and wall migration energy, which will be discussed later, are much smaller just below the Curie temperature than at 0 K, and (ii) the wall–wall interaction energy is negligible. This picture is consistent with the recent Landau theory result [14] that AP-only walls should decay into two AP+FE walls. On electric-field poling, which grows the domains of one ferroelectric orientation at the expense of the oppositely oriented domains, one might, therefore, expect that the thickness of the oppositely oriented domains should be reduced to this very small value. In contrast, however, Jungk et al. [16] measured using PFM that the width of oppositely polarized domains is 60±10 nm after electric-field poling and subsequent field removal. The origin of this discrepancy is unclear; in our energy minimizations, the AP-only and FE-only DWs never separate to yield larger regions of the intermediate phase AP+FE structure, because the weak interaction between DWs is not a strong enough driving force for them to separate from their initialized positions. Another possibile origin for the discrepancy between our first-principles calculations and this experimental result is domain reconstruction at the surface caused by the depolarizing field yielding a non-bulk domain structure at the surface. Comparison between theoretical calculations and experimental reports Recent STEM studies [17] of neutral AP+FE DWs, showed two distinct wall types for the related compound TmMnO 3 . One, which occurs in the bulk region of the sample, has Tm displacements consistent with our {210} ‘sharp’ DW structure. In order to see the correspondence it must be recognized that Fig. 3a of [17] has the opposite orientation from our calculated supercell. The second, which was observed only at the edges of the sample, is consistent with the model with one Y ion at the wall in its paraelectric position proposed by Choi et al. [15] , that we do not find to be the lowest energy structure. Next, we calculate explicitly the structure and energetics of such walls, by imposing twofold rotation and c -glide reflection symmetries during our structural optimziation; we refer to these walls as 2/ c models. Fig. 3d shows our calculated lowest energy walls within the constraints of the 2/ c symmetry for {120} and {210} DWs in a 300-atom supercell, and the calculated Mn-O distances, θ and φ angles, and local polarizations. We find that, after structural relaxation, only the constrained Y atom directly at the boundary retains its paraelectric position with the Y ions on either side adopting their bulk positions. In contrast to the sharp walls, the polarization drops to zero at the wall and the phase angle φ changes to 30°. This is reminiscent of the centrosymmetric InMnO 3 structure in which of the In ions retain six-coordinated high-symmetry positions and the MnO 5 bipyramids trimerize at angles intermediate to those of the YMnO 3 structure, φ =30°+ n ·60° [13] . As in the sharp wall case, the Mn-O distances remain constant across the wall, indicating that the MnO 5 bipyramids retain their shape, although their tilting magnitude is reduced, consistent with the smaller tilting magnitude in the structure (4.5°) compared with the P 6 3 cm (5.1°). Our calculated {120} 2/ c walls, in particular the pattern of Y displacements (down-down-up-middle-down-up-up from left to right through the wall), matches well the STEM results of Fig. 4 in [17] for the walls at the edges of the sample (Again the image has the opposite orientation from our calculated supercell). Our calculated average energy for the 2/ c DWs is high, however. We obtain a value of 195 meV/DW≈44.8 mJ m −2 by linearly extrapolating the values from four supercells each containing one {120} and one {210} DW, to infinite DW spacing. This is four times the value calculated for the fully relaxed walls. The occurence of this high-energy wall type concurrently with the lowest energy wall in the same sample remains to be understood, although it is possible that truncation of the electrostatic potential or defect accumulation at the edge of the sample modifies the energetics. DW migration In conventional ferroelectrics, the electric polarization is reversed on application of an electric-field through the migration of the DW. Next, we study a possible microscopic migration mechanism of the coupled AP+FE walls in YMnO 3 by calculating the energy landscape for DW migration, as well as the structure of the transition state using the nudged elastic band method [26] . In Fig. 6 we show our calculated energy landscape for migration of AP+FE walls in YMnO 3 , as well as the structure of the transition state. We find that the structure at the maximum of the migration energy curve, as well as the energy, are in fact those of the 2/ c DW. As the DW moves, the Y ions at the boundary move through their paraelectric positions, with the MnO 5 trigonal bipyramids rotating simultaneously to the 30° phase positions. The DW width increases from ~0 to 1 unit cell during the migration, as the DW moves from one side of the intermediate 2/ c structure to the other. The energy barrier height is 33.2 mJ m −2 , which is almost three times the DW energy. Although the barrier height is comparable with that of PbTiO 3 (37 mJ m −2 ), its ratio to the DW energy is much higher than that of PbTiO 3 , where the energy barrier is only 36% of the DW energy [22] . In addition, the polarization is an order of magnitude smaller in YMnO 3 than in PbTiO 3 , and thus the electric-field to move the walls through this mechanism should be correspondingly higher. Indeed, recently Skumryev et al. [27] have reported that, while ferroelectric hysteresis is observed at room temperature, it cannot be obtained at 5 K. As our DFT calculations are performed at 0 K, our calculated relatively higher migration energy with respect to the polarization compared with conventional ferroelectrics is consistent with this observation. However, while our proposed pathway is a plausible DW migration mechanism, we cannot make definitive statements about the domain switching mechanism. For further studies, finite electric-field calculations that allow us to directly simulate the DW migrations would be imperative. 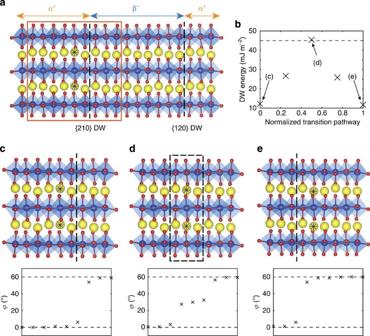Figure 6: Migration of DWs. (a) Initial structure for calculating the migration of a {210} AP+FE DW with nudged elastic band (NEB) method. (b) The calculated energy landscape through the DW migration. The dashed line indicates the average DW energies for 2/cmodels. (c–e) The initial, intermediate and final structures (upper panels), and trimerization phases (lower panels). As the DW moves, the Y ions indicated by the stars move through their paraelectric positions, with the MnO5trigonal bipyramids rotating simultaneously. Figure 6: Migration of DWs. ( a ) Initial structure for calculating the migration of a {210} AP+FE DW with nudged elastic band (NEB) method. ( b ) The calculated energy landscape through the DW migration. The dashed line indicates the average DW energies for 2/ c models. ( c – e ) The initial, intermediate and final structures (upper panels), and trimerization phases (lower panels). As the DW moves, the Y ions indicated by the stars move through their paraelectric positions, with the MnO 5 trigonal bipyramids rotating simultaneously. Full size image Topological defect Based on our finding that the lowest energy AP+FE DWs have the sharp configuration, in this last section we discuss the likely structure of the topological defects that form at the meeting points between six AP+FE DWs, Fig. 7a . From geometrical considerations, when six Y ions meet around a central point as in Fig. 7b , those in the α + , β + and γ + domains correspond to the same site in the unit cells of Fig. 2a (lower right say, with two up and one down), and those in the α − , β − and γ − correspond to the other site (say upper left, with two down and one up). The resulting pattern of up/down Y ion displacements—in which half displace up and half down along the z axis but not in an alternating pattern—is then shown in Fig. 7b . We see that the local symmetry at the topological defect is lower than those of both the bulk and the DWs. This pattern of displacements causes a frustration of the Y ion at the centre of the topological defect, which cannot displace in a direction that allows all DWs to maintain their sharp configuration. It is likely, therefore, that the Y ion at the centre remains at its paraelectric position; otherwise a modification of the wall structure would be required in the vicinity of the topological defect. We note that this picture does not correspond to that of [15] , which used the higher energy 2/ c models for the DWs meeting at the defect. It is clear that further theoretical and microscopy studies would be desirable for a full understanding of the structure of the topological defects. 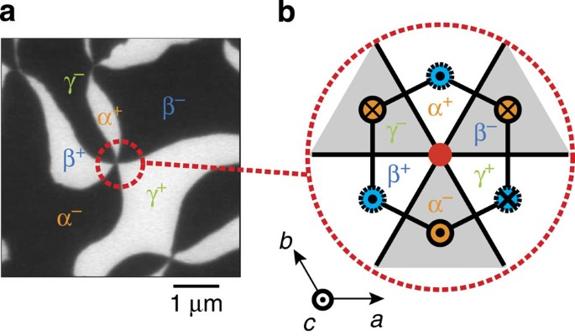Figure 7: Atomic structure around topological defect. (a) Domain pattern in YMnO3measured using PFM. (Reprinted with permission from13. Copyright (2012) by the American Physical Society. (b) One of the six possible equivalent sets of Y ion (blue and orange circles) displacements around the topological defect. Figure 7: Atomic structure around topological defect. ( a ) Domain pattern in YMnO 3 measured using PFM. (Reprinted with permission from [13] . Copyright (2012) by the American Physical Society. ( b ) One of the six possible equivalent sets of Y ion (blue and orange circles) displacements around the topological defect. Full size image We have used first-principles density functional theory to calculate the structure and properties of the low-energy structural DWs in the hexagonal manganites. We find that the lowest energy DWs are atomically sharp, with {210} orientation, explaining the orientation of recently observed stripe domains and suggesting their topological protection. We show that AP-only and FE-only DWs do not exist, but instead always have a finite intermediate thickness of AP+FE DW as observed experimentally. We determine the lowest energy pathway for ferroelectric switching through domain-wall motion and show that it occurs via the recently identified paraelectric InMnO 3 structure. Finally, we suggest a structure for the cores of the sixfold topological defects. Theoretical calculations First-principles spin-polarized calculations were performed using the projector-augmented wave method [28] as implemented in Vienna Ab initio simulation package (VASP) [29] . The exchange–correlation interactions among electrons were treated using the local density approximation with Hubbard U correction [30] , [31] . The parameters were set to the values of previous reports ( U =8 and J =0.88 eV on the Mn-3 d orbitals) [32] , and A -type magnetic configuration was adopted. Lattice constants for the calculation of DWs were fixed to the values of the relaxed unit cell without DWs, and internal positions were optimized in each case until the forces acting on all atoms converged to <0.005 eV Å −1 . We tested the convergence of the plane wave cutoff energy and k -point sampling ( Supplementary Fig. S3 ), and the effect of Hubbard U and magnetic configuration ( Supplementary Fig. S4 and Supplementary Note S2 ). The cell size dependence was checked by adopting supercells of several sizes containing up to 300 atoms. The visualization of crystal structures was performed with vesta [33] . How to cite this article: Kumagai, Y. et al. Structural domain walls in polar hexagonal manganites. Nat. Commun. 4:1540 doi: 10.1038/ncomms2545 (2013).